Impact tolerance in mussel thread networks by heterogeneous material distribution The Mytilidae , generally known as marine mussels, are known to attach to most substrates including stone, wood, concrete and iron by using a network of byssus threads. Mussels are subjected to severe mechanical impacts caused by waves. However, how the network of byssus threads keeps the mussel attached in this challenging mechanical environment is puzzling, as the dynamical forces far exceed the measured strength of byssus threads and their attachment to the environment. Here we combine experiment and simulation, and show that the heterogeneous material distribution in byssus threads has a critical role in decreasing the effect of impact loading. We find that a combination of stiff and soft materials at an 80:20 ratio enables mussels to rapidly and effectively dissipate impact energy. Notably, this facilitates a significantly enhanced strength under dynamical loading over 900% that of the strength under static loading. Dynamic loading can be treacherous for engineered and natural systems because the force is rate-dependent and can easily become extremely large, leading to catastrophic failure. For example, forces on a building’s pillars during earthquakes or explosions reach several times of that of its static weight. In the natural world, mussels attached to rocks or hulls of ships experience significant mechanical forces due to dynamical loading [1] , [2] , but thrive in this extreme mechanical environment. On the other hand, the strike force exerted by stomatopods (a species of marine crustaceans) reaches hundreds of Newtons, large enough to smash the shell of clams [3] . However, how to effectively design structures to diminish the damage caused by dynamic loading remains unanswered. Mussels have been cited as model systems for adhesives that facilitate strong attachments to wet surfaces ( Fig. 1a ) [4] , [5] , [6] , [7] , [8] , [9] , including stone, wood, concrete and steel, and are subjected to severe mechanical impacts caused by waves [1] , [2] . Indeed, earlier work has explored properties of dihydroxyphenylalanine as a key adhesion protein, found at the end of a byssus thread’s adhesion plaque ( Fig. 1b ) [4] , [6] , [7] , [10] , [11] , [12] , [13] . Unlike other species such as affixed barnacles, mussels dangle at a distance from the substrate and their connection is provided by the network of byssus threads. However, the static strength of the mussel attachment is much smaller than the force imposed by waves, owing to effects of dynamic loading that has been measured to exceed 250% of the static strength [2] . Fast moving ships and rocky shorelines are challenging environments, owing to high waves and fast moving water. In spite of these adverse conditions, hulls of ships and rocky shorelines are filled with mussels. 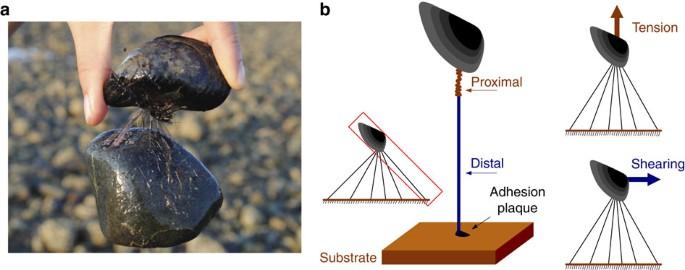Figure 1: The musselM. edulisand its byssus network. (a) Picture of a musselM. edulisattached to a rock, found at a rocky shoreline in the Boston area. (b) Schematics of the composition of the byssus network and the two loading modes (tension and shearing). Figure 1: The mussel M. edulis and its byssus network. ( a ) Picture of a mussel M. edulis attached to a rock, found at a rocky shoreline in the Boston area. ( b ) Schematics of the composition of the byssus network and the two loading modes (tension and shearing). Full size image Here we report the first detailed investigation of the mechanical behaviour and failure of marine mussel thread networks. To examine how mussels deal with adverse mechanical conditions, we use a method that combines experimental testing and computational modelling to systematically investigate how the material property of simple mussel threads affects its adhesion to rocks or ships. We analyse the failure of marine mussel attachment and demonstrate that the heterogeneous material distribution in byssus threads, with a combination of stiff and soft materials at an 80:20 ratio, enables them to decrease the effect of impact loading. This specific material design allows the greatest force reduction to mitigate the negative effects of dynamic loading. This peculiar material distribution facilitates a significantly enhanced dynamic strength of the attachment over 900% compared with the static strength, realized in an intriguing interplay of material and geometry that covers multiple length and time scales. Our investigation reveals the underlying reason for the remarkable properties of mussel adhesion, which rely on a particular heterogeneous distribution of stiff and soft materials in a particular architecture. The derived concept has implications beyond the specific case of mussel attachment, and advances our understanding of strategies of material design for impact tolerance and the design of attachment devices for broad applications in engineering. Tensile test and the static strength of byssus network In order to gain fundamental understanding of the global mechanical behaviour of the entire byssus network and its static strength, we assess the adhesion force between a clay substrate and the entire mussel ( Mytilus edulis ) using a tensile machine, for two loading modes, tension and shearing, in order to represent two extreme types of forces a mussel encounters ( Fig. 1b ). A series of snapshots of the deformation process of the byssus network under external loading is shown in Fig. 2a,c as well as corresponding force-extension curves depicted in Fig. 2b,d . Both force-extension curves feature two regimes before rupture, an initial linear regime and a subsequent stiffening regime. During the first regime, all byssus threads rotate towards the loading direction and more threads are subjected to tension. During the second regime, the elongation of aligned byssus threads contributes to the increasing strain, and the deformation of the soft proximal part is more significant than that of the stiff distal part. We repeat the measurements on different mussels similar in size and find strengths as 5.4±1.8 N (tension) and 5.1±2.8 N (shearing), where the measured force level agrees well with earlier test results [1] . The force is one order of magnitude larger than the mussel’s self-weight of 0.09±0.02 N without sea water between valves, or ~0.3 N with sea water between valves ( Supplementary Table S1 ), ensuring its attachment in air at low tide. Yet, the strength is much smaller than the dynamic impact force, which is defined as the mean value of instant dynamic loading generated from waves on the fixed mussel at shores (measured to be ~17.8 N [2] ). The impact force exceeds the strength of mussel threads and should make it impossible for the mussel to attach to bare rock, and make this an unlikely place to settle. However, this contradicts the observation that many isolated mussels are frequently found at exposed rocks and ships ( Fig. 1a and Supplementary Fig. S1 ). Considering the fact that the dynamic loading is much larger than the static strength of byssus threads, the mechanical function of the byssus thread is more than simply affixing the mussel to the environment. 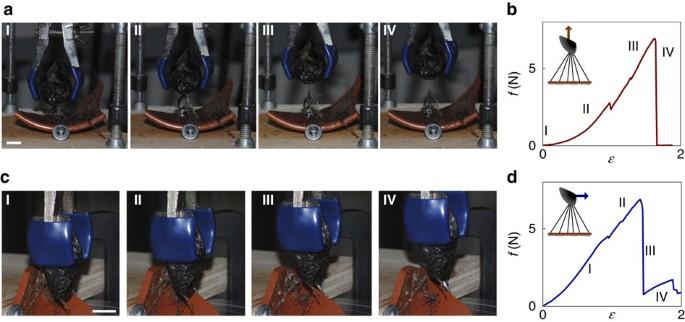Figure 2: Experiments and force-extension curves for the byssus network. (a) Snapshots of the byssus network under the tension mode loading. Snapshots I–IV are taken at applied strain of 0, 0.66, 1.39 and 1.64, respectively. Scale bar, 10 mm. (b) Force-extension (f–ε) curve of the network corresponds to the snapshots ina, with each corresponding strain noted in the plot. (c) Snapshots of the byssus network under the shearing mode loading. Snapshots I–IV are taken under the strain of 0.74, 1.09, 1.40 and 1.76, respectively. Scale bar, 10 mm. (d) Force-extension curve of the network corresponds to the snapshots inc, with each corresponding strain noted in the plot. Figure 2: Experiments and force-extension curves for the byssus network. ( a ) Snapshots of the byssus network under the tension mode loading. Snapshots I–IV are taken at applied strain of 0, 0.66, 1.39 and 1.64, respectively. Scale bar, 10 mm. ( b ) Force-extension ( f – ε ) curve of the network corresponds to the snapshots in a , with each corresponding strain noted in the plot. ( c ) Snapshots of the byssus network under the shearing mode loading. Snapshots I–IV are taken under the strain of 0.74, 1.09, 1.40 and 1.76, respectively. Scale bar, 10 mm. ( d ) Force-extension curve of the network corresponds to the snapshots in c , with each corresponding strain noted in the plot. Full size image Experiment-based computational modelling The mussel with the network of byssus threads forms a complex structure, in which the link between architecture of the structure and the material properties of the threads are coupled. To gain insights into the mechanical behaviour of the byssus network under loading, we model the byssus network based on our own experimental measurements and literature data, and use the model to carry out a series of computational experiments to understand the mechanisms by which it can successfully deal with severe mechanical conditions. We model each byssus thread as three parts with distinct mechanical properties, that is, the proximal part, the distal part and the adhesion plaque as illustrated in Figs 1b and 3a . The tensile properties of the first two parts are fitted to experimental measurements [1] as shown in Fig. 3b (details in the Methods section). Their differences are likely caused by the different ratio of secondary structures [14] , [15] . The umbrella-shaped byssus network model is built based on a single thread model with its shape described by the height–radius ratio ( H/R ). We model ten threads in the network as it is the maximum number of threads that deform together, which is interpreted from our own experiments, and as has been shown in literature [1] . For each thread of the length L , CL denotes the length of the distal part and (1− C ) L the length of the proximal part, where C =80% corresponds to the natural composition of the byssus thread [1] , [15] , [16] . Owing to the lack of knowledge about the interacting strength between the mussel foot protein and clay, we perform tensile tests for single threads as illustrated in Fig. 3c and Supplementary Fig. S2 , and obtain the detachment force as 0.4±0.1 N as shown in Fig. 3d . We also performed mechanical tests on several surfaces including natural rock and wood that are relevant to the substrates inhabited by mussels. We find that rocks yield a similar adhesion strength as clay. For wood, the strength fluctuates significantly as the wood substrate tends to rot in sea water. We combine these results to model each byssus thread (details in the Methods section and Supplementary Table S2 ) and apply tensile force to a single thread at the distal part in simulation to validate our model against experimental observations. Our model reproduces the experimental data well, and rupture occurs consistently at the plaque–substrate interface ( Fig. 3e ). The force-extension curve, as shown in Fig. 3f , is composed of a linear regime followed by a softening regime before failure at 0.4 N, in good agreement with experiments. These established agreements between simulation and experiment suggest that our model reflects the mechanical behaviour of byssus threads under loading. In addition to measuring the nonlinear elastic properties of the threads, we perform measurements to obtain the viscosity within a single byssus thread as shown in Fig. 4a–c (additional details provided in the Supplementary Method 1 ). This viscosity added to the particle interactions in the thread model yields a viscous force along the byssus thread. We test the mechanical responses of the thread under very different pulling rates and validate these results against experimental tensile tests under corresponding pulling rates [15] (as shown in Supplementary Fig. S3 ). We use this model to assess how viscosity affects the mechanical response of the byssus network. To do this, we deform the entire byssus network by using pulling rates from 1 m to 10 m s −1 and find that the viscosity term has a negligible effect on the force-extension curves, as shown in Fig. 4d . 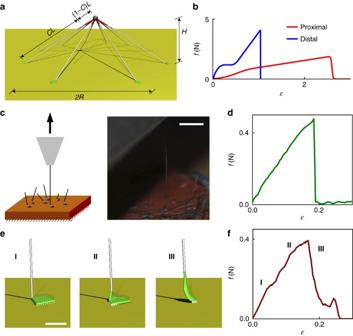Figure 3: Experimental and computational tests of a single thread. (a) Configuration and geometric characteristics of a byssus thread network model. The grey bead represents the centre of mass of the mussel. (b) Tensile property of the proximal part and the distal part of a single thread. (c) Schematic figure to illustrate how we test the single fibre’s adhesion force in experiment. Scale bar, 4 mm. (d) Force-extension curve of a single thread under tension obtained in the experimental tensile test. (e) Computational snapshots of the single thread under tension, fracture at the adhesion plaque governs the failure of the thread. Scale bar, 2 mm. (f) Computational result of the force-extension of the single thread model corresponds to the snapshots ine, with each corresponding strain noted in the plot. Figure 3: Experimental and computational tests of a single thread. ( a ) Configuration and geometric characteristics of a byssus thread network model. The grey bead represents the centre of mass of the mussel. ( b ) Tensile property of the proximal part and the distal part of a single thread. ( c ) Schematic figure to illustrate how we test the single fibre’s adhesion force in experiment. Scale bar, 4 mm. ( d ) Force-extension curve of a single thread under tension obtained in the experimental tensile test. ( e ) Computational snapshots of the single thread under tension, fracture at the adhesion plaque governs the failure of the thread. Scale bar, 2 mm. ( f ) Computational result of the force-extension of the single thread model corresponds to the snapshots in e , with each corresponding strain noted in the plot. 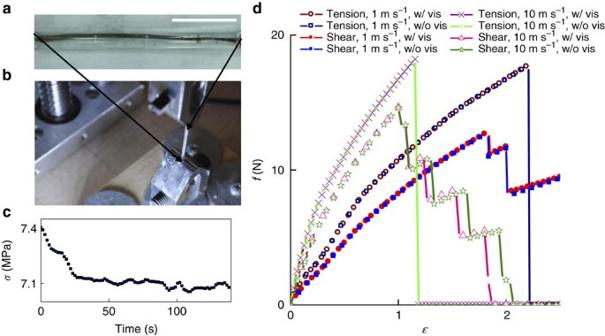Figure 4: Viscosity and mechanical response. (a) A mussel thread is kept in a thin tube (inner diameter, 0.6 mm) filled with sea water, scale bar, 4 mm. (b) The thread and tube is mounted on a tensile machine while the thread is in tension while the upper clamp moves at a constant strain rate of 0.02 s−1. (c) We slightly deform the thread to reach the stress (σ) of 7.4 MPa, stop loading and record the stress relaxation as a function of time. The residue stress converges at a 7.1 MPa level. (d) Simulation results of the force-strain curves of the byssus network under different pulling rates and modes. We test the model with a geometry as shown inFig. 3awith (w/) and without (w/o) considering the viscosity within a single thread. The model is stretched both in tension and shearing modes with 1 and 10 m s−1loading speeds (strain rate of 33 and 333 s−1), which are very relevant to the impact speeds (up to 3.5 m s−1) on mussels. Overlapping of the curves (with and without the viscosity term) before the peak force suggests that the viscosity term has a negligible effect on the mechanical response of the byssus network under loading. Full size image Figure 4: Viscosity and mechanical response. ( a ) A mussel thread is kept in a thin tube (inner diameter, 0.6 mm) filled with sea water, scale bar, 4 mm. ( b ) The thread and tube is mounted on a tensile machine while the thread is in tension while the upper clamp moves at a constant strain rate of 0.02 s −1 . ( c ) We slightly deform the thread to reach the stress ( σ ) of 7.4 MPa, stop loading and record the stress relaxation as a function of time. The residue stress converges at a 7.1 MPa level. ( d ) Simulation results of the force-strain curves of the byssus network under different pulling rates and modes. We test the model with a geometry as shown in Fig. 3a with (w/) and without (w/o) considering the viscosity within a single thread. The model is stretched both in tension and shearing modes with 1 and 10 m s −1 loading speeds (strain rate of 33 and 333 s −1 ), which are very relevant to the impact speeds (up to 3.5 m s −1 ) on mussels. Overlapping of the curves (with and without the viscosity term) before the peak force suggests that the viscosity term has a negligible effect on the mechanical response of the byssus network under loading. Full size image Dynamic response under impact loading Impact loading applied to the mussel is modelled as an instantaneous initial velocity of the mussel’s body, reflecting that it accounts for 99.5% of the total mass of the system. According to the experiment, the measured impact force of 17.8 N yields an instantaneous velocity of 2.0 m s −1 at the center of mass of the mussel where the byssus threads attach to (see the Methods section for details). We test the instantaneous velocity both in the vertical direction for the tension mode and along the substrate for the shearing mode, as shown in Fig. 5a,c , respectively. We find that the proximal part undergoes significant deformation as the mussel moves apart while the distal part remains in a relaxed state with zero tensile force. The tensile force in the proximal part is rather sensitive to the movement of the mussel from its equilibrated position as it reaches a peak within 0.01 s. However, the tensile force in the distal part at that moment is only halfway to reaching the peak force, as shown in Fig. 5b,d . The peak force in the distal part is much smaller than that of the proximal part, and reaches 80% in the tension mode and only 53% in the shearing mode. The proximal part connected to the mussel effectively buffers the impact to the adhesion plaque. Therefore, we can understand the role of the proximal part as a safety belt of the byssus network, as it is critical to absorb the impact loading. We increase the initial speed stepwise in the simulations, and find that the maximum impact speed for failure is 3.3 m s −1 for tension and 3.5 m s −1 for shearing. Those initial velocities correspond to a maximum impact force of 48.5 N, which is over nine times that of the static strength. This value agrees well with the highest impact forces on mussels that have been recorded at shores and reported in the literature [2] . 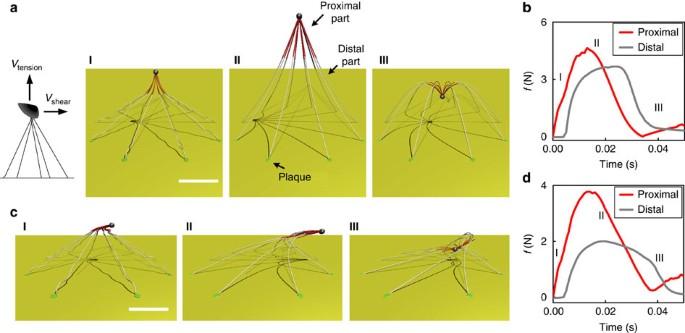Figure 5: Dynamic response of the byssus thread network after impact. (a) Simulation snapshots of the deformation of the byssus network under the impact loading by giving the mussel an initial velocity of 2 m s−1in the tension direction. Scale bar, 20 mm. (b) Sum of the force within the byssus threads at the proximal part and that at the distal part as functions of time for the tension mode. In this plot, we denote the time when each subfigures I to III inais taken in simulation. It is noted that the mussel stretched by the byssus network decelerates, and then moves in the opposite direction as shown in III. (c) Simulation snapshots of the byssus network under the impact loading by giving the mussel an initial velocity of 2 m s−1in the shearing direction. Scale bar, 20 mm. (d) Sum of the force within the byssus threads at the proximal part and that at the distal part as functions of time for the shearing mode. In this plot, we denote the time when each subfigure I to III incis taken in simulation. Figure 5: Dynamic response of the byssus thread network after impact. ( a ) Simulation snapshots of the deformation of the byssus network under the impact loading by giving the mussel an initial velocity of 2 m s −1 in the tension direction. Scale bar, 20 mm. ( b ) Sum of the force within the byssus threads at the proximal part and that at the distal part as functions of time for the tension mode. In this plot, we denote the time when each subfigures I to III in a is taken in simulation. It is noted that the mussel stretched by the byssus network decelerates, and then moves in the opposite direction as shown in III. ( c ) Simulation snapshots of the byssus network under the impact loading by giving the mussel an initial velocity of 2 m s −1 in the shearing direction. Scale bar, 20 mm. ( d ) Sum of the force within the byssus threads at the proximal part and that at the distal part as functions of time for the shearing mode. In this plot, we denote the time when each subfigure I to III in c is taken in simulation. Full size image Energy absorption and dynamical strength by structure In order to understand the underlying mechanism, and specifically how the material distribution in the byssus thread (that is, the ratio of stiff material versus the entire thread, here denoted by C ) is adapted to dynamic loading, we systematically alter the ratio between the distal and proximal parts and the geometry of the byssus network, and investigate how those characteristics affect the dynamic response of the byssus network under impact loading. The total energy of the system (the sum of kinetic energy and potential energy) as a function of time before the mussel reaches maximum deformation is shown in Fig. 6a,b for the tension and shearing modes, respectively. The energy dissipation for byssus threads with a proximal part is significantly higher than the byssus thread composed of a pure distal part ( C =1). We measure the time when the total energy decreases to half of its initial value as shown in Fig. 6c,d , where C =1 corresponds to the slowest total energy dissipation while decreasing C corresponds to faster energy dissipation. The transition between C =0.5 and 1 contributes mostly to the increment of the rate of energy dissipation. We repeat the measurement of the decay time of the kinetic energy to its half value ( Fig. 6c,d and Supplementary Fig. S4 ) and find that a larger C leads to a greater advantage in terms of its ability to decrease the kinetic energy. This shows that the combination of those two materials benefits the energy absorption of the byssus network as the distal part quickly transits the instant kinetic energy into potential energy, while the proximal part dissipates the kinetic energy by viscosity. For pure elasticity, the peak force is proportional to where K eff is the effective stiffness of the network and m is the mass of the mussel while for pure damping the peak force is proportional to vη eff where η eff is the effective coefficient of viscosity, which depends on the thread diameter and the value of water viscosity. 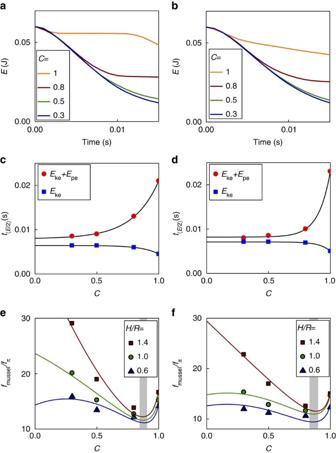Figure 6: Composition and structure affect the energy and force. (a,b) History of the total energy (E) of the byssus network under impact loading before the maximum displacement of the mussel. (c,d) Time constants () when the kinetic energy (Eke) and the total energy (as the sum ofEkeand potential energy (Epe) asE=Eke+Epe)decrease to half of their initial values. Continue curves are obtained by exponential fit. The results summarized in (a–d) are for the byssus network withH/R=0.6. (e,f) Normalized reaction force, given by the ratio of the peak force exert to the mussel (fmussel) and the maximum peak force on the adhesion plaque (fπ), is shown for differentCandH/Rof the network. The continue curves are fitted results as given by equation (8) (with parameters summarized inSupplementary Table S3). For eachH/R, theCvalue that gives the minimum force is coloured in grey in the graph.a, candeare results of the tension mode, andb, dandfare results of the shearing mode. The reaction force experienced by the mussel is proportional to (detailed derivation in the Methods section) Figure 6: Composition and structure affect the energy and force. ( a , b ) History of the total energy ( E ) of the byssus network under impact loading before the maximum displacement of the mussel. ( c , d ) Time constants ( ) when the kinetic energy ( E ke ) and the total energy (as the sum of E ke and potential energy ( E pe ) as E=E ke +E pe )decrease to half of their initial values. Continue curves are obtained by exponential fit. The results summarized in ( a – d ) are for the byssus network with H/R =0.6. ( e,f ) Normalized reaction force, given by the ratio of the peak force exert to the mussel ( f mussel ) and the maximum peak force on the adhesion plaque ( f π ), is shown for different C and H/R of the network. The continue curves are fitted results as given by equation (8) (with parameters summarized in Supplementary Table S3 ). For each H/R , the C value that gives the minimum force is coloured in grey in the graph. a, c and e are results of the tension mode, and b, d and f are results of the shearing mode. Full size image We compute the reaction force exerted on the mussel from the proximal part ( f mussel ) normalized by the peak force recorded for the adhesion plaque ( f π ) as shown in Fig. 6e,f and fit the data according to equation (1) (details in the Methods section). The critical C value to minimize the reaction force is obtained at C =0.8~0.9, which agrees with the naturally existing percentage of the distal (~80% [1] , [15] , [16] ) and proximal part (~20% [1] , [15] , [16] ). The material distribution governs the viscoelasticity of the entire byssus thread network, and as shown by our data ( Fig. 6e,f ), this critical distribution yields a minimum reaction force on the mussel before detachment occurs. This critical value is not sensitive to the water viscosity as C =0.92 is obtained for water with larger viscosity (150% that of the room temperature at 10 °C) and C =0.74 is obtained for water with small viscosity (63% that of the room temperature at 50 °C). This is the most important result of our analysis, suggesting that the naturally observed distribution of two distinct materials (stiff and soft) leads to the least force at the junction between mussel and byssus threads, through a coupled mechanism in which material distribution and architecture work together for the benefit of the entire system behaviour. This result is found universally for varied geometries as H/R is changed from 0.6–1.4. Moreover, a smaller ratio of H/R induces an even smaller force and this finding, combining with the lower wave speed due to the no-slip condition of fluids closer to the substrate, enhances the mussel’s adaption to different environments. The composition and arrangement of the byssus threads leading to the least force at the proximal part under impact loading makes the mussel’s adhesion distinct from spider web anchorages. This difference is traced to the different biological functions of the two structures. Byssus threads connect directly to the mussel’s tissue and they need to avoid extremely large forces that may harm the tissue, while the spider web’s anchorage has a primary role in maximizing the adhesion force [17] . The few and thin byssus threads that mussels use to affix themselves to the environment provides them with significant lack of restrictions for feeding and migration in order to cope with environmental changes. According to our results, direct impacts with speeds lower than 3.3 m s −1 (~12 km h −1 ) to the mussel are safe for the byssus network. Because of the affinity of the mussels to the substrate, the flow speed around the mussel never exceeds 10% of the free-stream velocity [18] , [19] . Thereby, the mussel can remain attached to the sea bottom or hulls of ships of up to 120 km h −1 surface wave speeds (or ship speeds), explaining how mussels survive and thrive in such extreme conditions. Many natural materials are known to generate advanced functions by refining their hierarchical structures over many length scales [20] , [21] , [22] , [23] . Here, we have shown in opposition to prevalent thinking, the remarkable properties of mussel adhesion networks are not due to the strength of the adhesion pads. Rather, they rely on a clever distribution of materials in a unique architecture. The novel mechanism reported here, in which the material distribution in the byssus thread decreases the reaction force experienced by the tissue owing to mechanical loading caused by waves or the motion of a ship, has implications far beyond the specific case of mussel adhesion as the design can be immediately applied in developing engineered adhesive systems that are subject to dynamic loading. Moreover, the tensile force exerted by the proximal part efficiently decelerates the mussel speed in a short time span, in order to prevent the mussel from high velocity detachment and colliding with rocks. These advanced characteristics guarantee that the byssus thread acts as a synergistic interfacial material with functions beyond serving merely as a ‘strong glue’. Interestingly, the principle of material distribution design has also been exposed in the stomatopod dactyl club [3] , as well as in ancient fish armour [24] . The structural and mechanical lessons gained by investigating the byssus network could provide us with important design principles that can be applied in the fabrication of interfacial materials that can function effectively under dynamic loadings, such as attachments to ships, submarines, in wind turbines, or for applications in space technologies [4] , [25] , [26] . From a slightly different perspective, we have found that the use of about 20% soft material in mussel threads is crucial in light of impact absorption and force reduction for the entire animal. This result is reminiscent of the Pareto principle [27] (also known as the 80/20 rule), given the fact that a tiny amount of causes account for almost all of the effects. This principle reflects the finding that the greatest force deduction comes from the soft material, which makes up only a small portion of the overall thread ( Fig. 1b ) [1] , [15] , [16] . This is a rule of thumb that has wide applications in social sciences, economics and business because it provides the empirical outcome of the balance between two competing mechanisms generally regarded as cost and gain. It is noted that this analogy is a conjecture at this point and that caution needs to be taken in the comparison. The agreement between the observation in mussel and the Pareto principle indicates that the design of byssus threads may reflect an optimal state of the competition between energy dissipation and thread deformation. Nature features an interesting repertoire of building materials, selecting the appropriate material and structure for distinct purposes. Here we find that, the remarkable properties of mussel adhesion are not merely owing to the strength of the adhesion pads, but rather rely on a specific distribution of stiff and soft materials in a unique geometry. This concept identified here is derived from an attachment system but has implications beyond this specific application, and provides a general advance in the understanding of mitigation strategies for impact loading. Hence, it could be applied in the design of attachments and implants in bioengineering, structural engineering and architecture, bio-inspired material design and polymer science. Mussel sample preparation and experimental setup The samples of M. edulis were collected in the native environment of Boston harbour area together with substrates made of clay. The cage was kept under sea for 3 weeks to ensure the mussels’ attachment. We carefully cleaned the samples with sea water before further testing the adhesion between the mussel and the substrate. The tensile tests were carried out in room temperature with a standard tensile testing machine (MTS Corporation, Eden Prairie, MN, USA). In each of the tensile tests, the substrate was clamped to the cross head, which moved at a constant rate of 0.1 mm s −1 displacement. The attached mussel was held by a force transducer where the reaction force was measured. The cross head displacement is measured using a linear voltage displacement transducer mounted inside the actuator. The total force applied to the mussel and the total displacement of the substrate were scanned with 1 Hz and saved to the connected data collector. Each sample was kept in a sea water tank before performing the test. Application of impact loading We apply an initial instant speed to the mussel to model the result of impact loading. The relevant velocities are converted from the in situ force history measured at shores. The impact force of is measured as the reference force at shore [2] , taking the force signal as general sinusoidal wave, the peak force equals . Considering the tethered Dacron string as pure elastic, the initial speed v 0 can thus be estimated by , where m is the weight of the mussel model and k is the elastic constant of the Dacron string. The values of those parameters used in the in situ force measurement study are m =0.045 kg and k =9,600 N m −1 for the 130 lbs string (consider 30% extensibility, 20 cm in length) [2] . This string has been used to tether between the mussel and force sensor to carry out the in situ measurements [2] . Those parameters yield an initial velocity of 2 m s −1 of the mussel model. The initial speed of 3.5 m s −1 is the maximum for our model before it starts to rupture. According to f p — v 0 relationship, this maximum initial speed yields to an impact loading of f p =48.5 N. This value agrees well with the highest impact forces on mussels that is recorded and reported in the literature [2] . Computational model of the byssus thread Each byssus thread is modelled by three segments: the proximal part, distal part and adhesion plaque ( Fig. 1b ). We use a simple bead-spring model to model the proximal and distal part with a diameter of d =250±40 μm as given by the experimental measurement ( Supplementary Fig. S2 ). This result agrees with the earlier measurement of byssus thread diameter in literature (275 μm for M. californianus [1] ). We use the tensile force-strain response of a single thread at different regions as measured experimentally in literature to define the nonlinear stiffness of the spring in tension [1] . Each of the stress–strain curves is composed of three regimes: elastic, yielding and post-yielding. We design the spring stiffness accordingly by using a multi-polynomial potential for the springs. The equilibrated spring length is r 0 =1 mm while the axial force under deformation is given by: where In equation (3), k i and r i are spring constants that derived directly from the force-extension curve of the experimental tensile test of the byssus thread at different regions. The Fermi–Dirac distribution function introduces two additional parameters r b and Ξ [28] . The parameter r b denotes the critical separation distance for breaking of the filament and the parameter Ξ describes the amount of smoothing around the breaking point (the smaller Ξ, the smoother the curve becomes). The parameters R 1 = H φ ( r = r 1 )= k 1 ( r 1 — r 0 ) and R 2 are calculated from force continuity conditions. H φ is the Hermite interpolation function that is used to smoothly connect the two linear curves [29] , which is defined as: Where m i and n i are coefficients determined by the connectivity conditions as H φ ( r=r 1 )= R 1 , H φ ( r = r 2 )= R 2 , H φ ′ ( r=r 1 )= k 1 and H φ ′ ( r=r 2 ) =k 2 and hence their values are given by An angular spring between two neighbouring springs is used to define the bending stiffness of the thread, and it is given by where E =4 k 1 r 0 /(π d 2 ) is the Young’s modules of the thread with different values for the two materials. The bending energy of each angular spring is φ B ( θ )=K B ( θ — π ) 2 , where θ is the angle between two neighbouring springs. Damping effects are included in the model by considering the energy dissipation of each byssus thread in motion caused by the viscosity of water environment. Because of the small dimension of the byssus thread, we use the Stokes’ law to measure the drag force by [30] : where μ =8.6 × 10 −4 Pa s is the fluid viscosity constant of water at room temperature and R is the equivalent spherical radius of the mesoscopic bead, which equals to the radius of a sphere of equivalent volume [31] . The parameter v denotes the relative velocity of particle motion in water. The numerical values of all the parameters for the model are summarized in Supplementary Table S2 . The adhesion plaque is modelled by a rectangular elastic network. The measurement results in a plaque size of l × l =1.9 × 1.9 mm 2 as shown in Supplementary Fig. S2 . The entire network is composed of n =100 beads, leading to the lattice length as . We use the density and Young’s modulus of the distal part to model the stiffness of the adhesive plaque. Considering that the plaque thickness equals to the thread diameter, the mass of each plaque bead is and the stiffness . The angular term of the plaque network is determined by the bending stiffness of the network in the two main axis as K B = Ed 3 /24. The adhesion strength between the plaque and the substrate is modelled according to the single-thread tensile result. For each adhesion point, the strength is given by , where F =0.4 N is the average strength of a single thread. The adhesion energy can be estimated by γ = nfδ / l 2 where δ =30 Å is the detachment distance as has been experimentally measured [7] . The result yields to 3.3 mJ m −2 , which agrees to mussel foot protein interaction strengths on mica measured by the surface forces apparatus [10] . Reaction force on the mussel The effective stiffness of the network is computed by where k distal and k proximal are the unit length stiffness of the distal part and the proximal part. The effective coefficient of viscosity is given by η eff = η distal C + η proximal (1− C ) where η distal and η proximal are the viscosity of the distal part and the proximal part. The reaction force applied to the mussel is thereby expressed as where a is a factor that measures the ratio of the contributions of the two forces to the total reaction force on the mussel. It has the physical meaning to measure how an elastic force increment relates to the increment of the total reaction force. We note that this parameter is different from C , which gives the ratio between two portions of a single thread but does not account for the network structure. The stiffness for the two parts is known as we used for modelling as k 1 as summarized in Supplementary Table S2 while η distal , η proximal and a are unknown factors in this function. It is noted that η distal and η proximal are not the viscosity of single byssus thread per se, as their values also relate to the structure of the network ( R and H here). The value of a also depends on the network structure. For the data points shown in Fig. 6e,f , we test each structure (with fixed R and H ) with different C , and take η distal , η proximal and a as parameters and determine their values by fitting. We use this function to fit the simulation results of the normalized reaction force on the mussel and obtain the continuous curve as shown in Fig. 6e,f . The fitting results and the critical C that leads to minimum reaction force are summarized in Supplementary Table S3 . The overall value of a is very close to unity, suggesting that both forces are equally important. Moreover, its value increases for larger H/R , indicating that the elastic force becomes slightly more dominating for a narrower and longer network (as its geometry turns from an opened umbrella into a closed one). How to cite this article: Qin, Z. & Buehler M. J. Impact tolerance in mussel thread networks by heterogeneous material distribution. Nat. Commun. 4:2187 doi: 10.1038/ncomms3187 (2013).